Correlating hydrogen oxidation and evolution activity on platinum at different pH with measured hydrogen binding energy The hydrogen oxidation/evolution reactions are two of the most fundamental reactions in distributed renewable electrochemical energy conversion and storage systems. The identification of the reaction descriptor is therefore of critical importance for the rational catalyst design and development. Here we report the correlation between hydrogen oxidation/evolution activity and experimentally measured hydrogen binding energy for polycrystalline platinum examined in several buffer solutions in a wide range of electrolyte pH from 0 to 13. The hydrogen oxidation/evolution activity obtained using the rotating disk electrode method is found to decrease with the pH, while the hydrogen binding energy, obtained from cyclic voltammograms, linearly increases with the pH. Correlating the hydrogen oxidation/evolution activity to the hydrogen binding energy renders a monotonic decreasing hydrogen oxidation/evolution activity with the hydrogen binding energy, strongly supporting the hypothesis that hydrogen binding energy is the sole reaction descriptor for the hydrogen oxidation/evolution activity on monometallic platinum. Hydrogen oxidation and evolution reactions (HOR/HER) are two of the key processes in renewable energy conversion and storage devices, including low-temperature fuel cells, which convert the chemical energy in hydrogen into electricity, and electrolysers, which store energy in chemical form by generating hydrogen from water. The state-of-the-art electrocatalyst for the HOR/HER is platinum (Pt) [1] , [2] . The rational design of HOR/HER electrocatalysts relies on a thorough understanding of the reaction mechanisms, and has been the research subject in both electrocatalysis studies and H 2 energy utilization [3] , [4] , [5] . The HER, as the probe reaction, has been widely investigated to elucidate the nature of the reaction intermediate [6] , [7] , as well as the correlation between reaction kinetics and metal surface properties [8] , [9] , [10] . Recent studies combining density functional theory (DFT) calculations and experimental data also demonstrate that the HER kinetics in terms of exchange current density in both low- and high-pH regimes correlate to DFT-calculated hydrogen binding energies (HBEs) via a volcano relationship, indicating that HBE can be used as the reaction descriptor for the HER [2] , [11] . Many types of efficient electrotrocatalysts have been developed including Pt-group metal-based alloys [12] , transition metal phosphides [13] , [14] , chalcogenides [15] , [16] , carbides [17] and even metal-free catalysts [18] . The knowledge acquired from the HER can be applicable to the HOR in terms of exchange current density. However, it is desirable to gain deeper understanding on the reaction rate on applied positive overpotential, that is, HOR reaction mechanism. Nevertheless, the extremely fast reaction kinetics of the HOR on Pt in low pH values make the quantification almost impossible with conventional electrochemical analytical techniques such as the rotating disk electrode (RDE) method [19] , [20] , by which true reaction kinetics are concealed by H 2 mass transport limitation. To resolve this problem, ‘H 2 -pump’ configuration in strong acidic polymer electrolyte environment has been adopted [21] , which minimizes the H 2 mass transport limitation. In comparison, the HOR/HER rates on Pt in base are drastically decreased, and can be quantified in high pH liquid electrolytes [19] . Durst et al . [22] studied the HOR/HER activities on carbon supported Pt, Pd and Ir nanoparticles (NPs) in both acid and base and found that the HOR/HER activities are approximately two orders of magnitude lower in base, but in both cases the reaction mechanism is the same with the Volmer step (discharging of adsorbed H) being rate limiting. However, there has been debate as to the reaction mechanism of the HOR in base. A bifunctional mechanism has been proposed, which involves the participation of adsorbed OH in the oxidation of H 2 (refs 20 , 23 ), while Durst et al . find that the HBE values acquired from cyclic voltammograms (CVs) in strong acid are smaller than those in strong base, and ascribe the slower HOR/HER kinetics in base to the stronger HBE. This hypothesis is supported by the larger discharging resistance for underpotentially deposited hydrogen (H UPD ) in base than in acid from impedance measurements [22] , suggesting that the HBE value should be the main reaction descriptor. Existing studies on the HOR/HER are mainly limited in the extremely low and high pH, which of course are relevant to the application of both proton and hydroxide exchange membrane fuel cells and electrolysers. However, an HOR/HER reaction rate difference as large as two orders of magnitude between strong acid and strong base suggests that an evolution of the reaction rate in the intermediate pH regime may exist. Thus, the HOR/HER in intermediate pH electrolytes, which has not been widely investigated, should shed light on the HOR/HER mechanisms. Moreover, previous correlations between the HER activity and metal surface properties are constructed on either gas phase H adsorption energy [8] or DFT-calculated HBE values [2] , [11] , the former of which may not be directly applicable to the electrochemical environment, while the latter does not incorporate the influence from water or H + /OH − in the electrolytes. Experimentally measured HBE values under electrochemical conditions are therefore desired to elucidate the mechanisms under reaction conditions. In this paper, we evaluate the HOR/HER polarizations and CVs of Pt in a wide range of pH ranging from 0 to 13. The monotonically decreased HOR/HER activities correlate well with the continuously strengthened electrochemical HBE values, strongly supporting the hypothesis that HBE is the sole reaction descriptor of the HOR/HER kinetics. HOR/HER on Pt in buffer solutions with pH from 0 to 13 Previous studies of the pH effects on the HOR/HER have been performed in both pH-buffered and unbuffered electrolytes of intermediate pHs using the RDE method, and show completely different behaviours [20] , [24] , [25] . If an unbuffered electrolyte is used, as protons are generated or consumed during the HOR/HER processes, the pH value at the Pt electrode surface will deviate from the bulk value, and in turn alter the intrinsic behaviour of Pt in the HOR/HER [24] , [25] . In our study, 0.2 M buffer capacity has been chosen as it can sufficiently mitigate the surface pH swing during the HOR/HER [24] , [25] . This is also confirmed by the lack of the plateau regions in the steady-state HOR/HER polarization curves ( Fig. 1a , see Supplementary Fig. 1 for the HOR/HER polarization curves of Pt in all investigated electrolytes), which would have appeared if an unbuffered or insufficiently buffered electrolyte was used [20] . The plateaus at 2–3 mA cm −2 disk in the HOR branch ( i lim ) are caused by limited H 2 transport to the electrode surface from the bulk electrolyte at a rotating speed of 1,600 r.p.m. ( ω in r.p.m.). 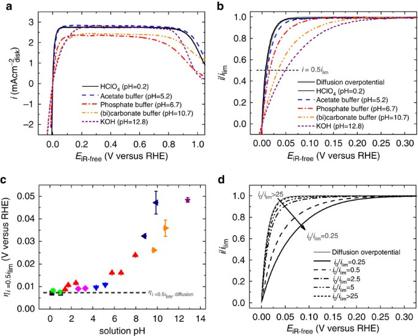Figure 1: HOR on Pt in a full range of solution pH and modelled HOR polarization curves. (a) Steady state positive-going sweeps of HOR polarization curves of Pt collected in selected H2-saturated buffer solutions. The sweep rate is 10 mV s−1and the rotating speed is 1,600 r.p.m. The polarization curves have been corrected for solution resistance. (b) HOR polarization curves normalized to the maximum limiting current densityilim. (c) Half-wave potential of the HOR in all pH-buffered electrolytes. Error bars are s.d. of at least two sets of experimental repeats. Black squares, perchloric acids (0.1 and 1 M); green circles, sulfuric acids (0.1 and 1 M); red up-triangles, phosphoric acid (0.1 M) and phosphate buffers; blue down-triangles, acetate buffers; magenta diamonds, citrate buffers; navy left-triangles, borate buffers; orange right-triangles, (bi)carbonate buffers; and purple stars, potassium hydroxide solution (0.1 M). Identical colour schemes are used for symbols in other figures. (d) Modelled HOR polarization curves using equations (2)–(4), , . The variation in the H 2 -limiting current density ( i lim ) is attributed to the different H 2 concentration ( ) and H 2 diffusivity ( ) in the electrolytes, and the different kinetic viscosity ( ϑ ) of the electrolytes, related by the Levich equation (equation (1)) [26] , Figure 1: HOR on Pt in a full range of solution pH and modelled HOR polarization curves. ( a ) Steady state positive-going sweeps of HOR polarization curves of Pt collected in selected H 2 -saturated buffer solutions. The sweep rate is 10 mV s −1 and the rotating speed is 1,600 r.p.m. The polarization curves have been corrected for solution resistance. ( b ) HOR polarization curves normalized to the maximum limiting current density i lim . ( c ) Half-wave potential of the HOR in all pH-buffered electrolytes. Error bars are s.d. of at least two sets of experimental repeats. Black squares, perchloric acids (0.1 and 1 M); green circles, sulfuric acids (0.1 and 1 M); red up-triangles, phosphoric acid (0.1 M) and phosphate buffers; blue down-triangles, acetate buffers; magenta diamonds, citrate buffers; navy left-triangles, borate buffers; orange right-triangles, (bi)carbonate buffers; and purple stars, potassium hydroxide solution (0.1 M). Identical colour schemes are used for symbols in other figures. ( d ) Modelled HOR polarization curves using equations (2)–(4), , . Full size image where n is the number of electrons transferred and F is the Faraday’s constant. Figure 1b provides a clearer demonstration of how the reaction kinetics changes with pH by normalizing the HOR current densities to the corresponding maximum plateau value i lim . The starting point of the HOR plateau shifts positively by 0.2 V from the 1 M HClO 4 solution (pH=0.2) to the 0.1 M KOH solution (pH=12.8), suggesting decreasing reaction rates with solution pH. The HOR current in HClO 4 (pH=0.2) solution appears to be completely under the H 2 mass transport limitation as pointed out in an early study [19] , assuming infinitely fast reaction kinetics [27] , [28] , according to where η diffusion is the diffusion-controlled overpotential and i d is the H 2 diffusion-limited current density (grey line in Fig. 1b ). In the HOR polarization curves, half-wave potential, defined as the HOR overpotential at i =0.5 i lim , also shows the same trend of the HOR with pH ( Fig. 1c ). When the pH<6, the apparent half-wave potentials are clustered around the diffusion half-wave potential of 9 mV (calculated using equation (2) with i d =0.5 i lim ). The seemingly ‘constant’ half-wave potential in pH<6 should not be interpreted as constant HOR activity in this pH regime, and it only suggests that the HOR in pH<6 is sufficiently fast so that the reaction is completely under H 2 mass transport control. As the solution pH goes above 6, the half-wave potential monotonically increases with the pH, indicating a continuously decreased reaction rate. It is noted that the half-wave potential in pH>6 should not be treated as the pure kinetic parameter as it includes both kinetic overpotential and H 2 diffusion overpotential due to the limitation using the RDE method, where H 2 mass transport is constrained. However, by normalizing the HOR currents to their limiting currents in different electrolytes, HOR in each electrolyte has the same diffusion overpotential (grey line in Fig. 1b ); thus the trend generated using half-wave potential as the activity indicator in this pH regime is valid as it contains the same diffusion overpotential. The exchange current densities ( i 0 ) in very strong alkaline environment such as the 0.1 M KOH solution (pH=12.8) and the bicarbonate/carbonate buffer (pH=10.7) are obtained by calculating the kinetic current density ( i k ) using the Koutecky–Levich equation (equation (3)) and then fitting to the Butler–Volmer equation where A rf is the roughness factor, defined as the ratio between the electrochemical surface area and the geometric area of the disk, α is the transfer coefficient and η is the overpotential. The exchange current density for 0.1 M KOH is determined to be 0.53 mA cm −2 Pt ( α =0.51), in excellent agreement with previous studies [19] , [22] . The exchange current density for the bicarbonate/carbonate buffer solution (pH=10.7) is slightly larger (0.63 mA cm −2 Pt ) and the transfer coefficient is ~0.6. Due to the fact that the HOR polarization curves in near neutral solutions are very close to the diffusion overpotential, it is not practical to extract accurate kinetic information including exchange current density and Tafel slope from the experimental polarization curves using the Koutecky–Levich equation, because close values of i and i d would cause significant uncertainty when extracting i k . Nevertheless, the exchange current density monotonically decreases with increasing half-wave potential as shown in Supplementary Fig. 2a ( Supplementary Note 1 for derivation). The most steep drop takes place in a very narrow range slightly above the half-wave potential (9 mV) constrained by the H 2 diffusion. The half-wave potential was then used to roughly estimate the exchange current density to obtain a better demonstration of the reaction kinetics. Supplementary Fig. 2b shows two orders of magnitude difference in exchange current density from pH=0 to 13. The polarization curves are further modelled by calculating current density ( i ) using equations (2)–(4), , , integrating the diffusion overpotential (2) and kinetic overpotential (4). As the reaction rate decreases ( i 0 / i lim decreases), the polarization curves deviates from the diffusion overpotential ( Fig. 1d ). The HER polarization curves of Pt in selected buffer solutions are shown in Fig. 2a , and the overpotential η at an HER current density of −1 mA cm −2 disk is compared in Fig. 2b . Similar to the HOR, the HER activity also decreases with increasing solution pH. The overpotential to reach an HER current density of −1 mA cm −2 disk changes from −3 mV for the pH=0 solution to −20 mV for pH in the range of 10–13. Unlike the HOR, where H 2 mass diffusion plays a role in the overall current, there is no limitation in H + transport in the HER. Therefore, the HER overpotential reflects the true kinetic information. 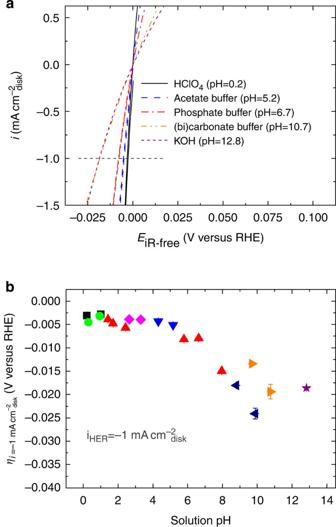Figure 2: HER on Pt in a full range of solution pH. (a) Steady state positive-going sweeps of HER polarization curves of Pt collected in selected H2-saturated buffered electrolytes. The sweep rate is 10 mV s−1and the rotating speed is 1,600 r.p.m. The polarization curves have been corrected for solution resistance. (b) Overpotential of the HER of Pt at a current density of −1 mA cm−2diskin all pH-buffered electrolytes. Error bars are s.d. of at least two sets of experimental repeats. Figure 2: HER on Pt in a full range of solution pH. ( a ) Steady state positive-going sweeps of HER polarization curves of Pt collected in selected H 2 -saturated buffered electrolytes. The sweep rate is 10 mV s −1 and the rotating speed is 1,600 r.p.m. The polarization curves have been corrected for solution resistance. ( b ) Overpotential of the HER of Pt at a current density of −1 mA cm −2 disk in all pH-buffered electrolytes. Error bars are s.d. of at least two sets of experimental repeats. Full size image HBE of Pt in buffer solutions with pH from 0 to 13 Unlike the HOR/HER results obtained in unbuffered electrolytes, where the reaction kinetics is concealed by the surface pH swing, the HOR/HER activities in buffered electrolytes clearly show a pH-dependent behaviour. To reveal the potential principle that governs the pH-dependent HOR/HER activities, surface properties of Pt, especially HBE values, have been examined under the same electrochemical conditions using cyclic voltammetry. 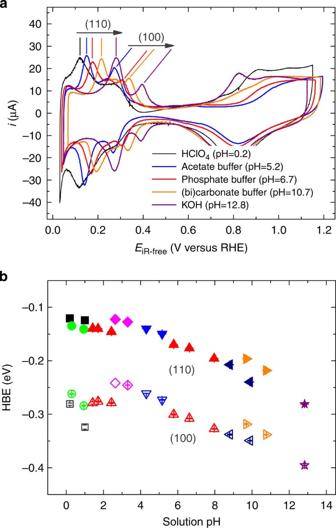Figure 3: CVs and HBEs of Pt in a full range of solution pH. (a) Steady state CVs of Pt collected in selected Ar-saturated electrolytes at a sweep rate of 50 mV s−1. The CV curves have been corrected for solution resistance. (b) HBEs on Pt(110) (solid symbols) and (100) (empty symbols) surfaces obtained from CVs as a function of solution pH. Error bars are s.d. of at least two sets of experimental repeats. Figure 3a shows the CVs of Pt in selected buffered electrolytes with solution pH ranging from 0 to 13 (see Supplementary Fig. 1 insets for the CVs of Pt in all investigated electrolytes). All of the CVs show well-defined i–E features of Pt including hydrogen adsorption/desorption (H UPD ) below ~0.5 V versus reversible hydrogen electrode (RHE), OH anion adsorption/desorption above ~0.6 V and a double layer region in between [29] . The peak at lower potential in the H UPD region corresponds to the H adsorption/desorption at the Pt(110) surface region (weakly bonded H), and the one at higher potential relates to the same process at Pt(100) (strongly bonded H) [29] , [30] . Both peaks shift positively by ~0.15 V when the solution pH changes from 0 to 13. As adsorption/desorption peak potential ( E peak ) directly reflects the HBE of Pt as in − FE peak =Δ H (ref. 31 ) (see ref. 31 and Supplementary Note 2 for derivation), the linear relationship between the HBE values ( E peak ’s taken from CVs collected in various buffer solutions) and the solution pH suggests that the HBE increases with increasing pH ( Fig. 3b ). The slopes are roughly −10 meV per pH for Pt(110) and −8 meV per pH for Pt(100), in good agreement with Koper’s studies performed in all phosphate buffer solutions with pH from 2 to 12 (refs 30 , 32 ). Note that the H desorption peaks on Pt(100) in strong acids, especially HClO 4 are usually very broad, leading to the difficulty in determining the precise adsorption energy. The slope is determined to be −12 meV per pH without the data in strong acids. It is noted that the HBE versus pH relation in our study is slightly more scattering compared with similar study performed in all phosphate buffer solutions [30] , [32] . To examine the potential anion effects on the HBE, CVs have been taken in 0.1 M KOH solution with the addition of KClO 4 and K 2 SO 4 salts, because ClO 4 − is known as a non-adsorbing anion, while SO 4 2− is a known strongly adsorbing anion, and the addition of these salts does not change the solution pH. Supplementary Fig. 3 shows that addition of SO 4 2− slightly changes the HBE of Pt (110) in 0.1 M KOH by less than 10 meV, while ClO 4 − has no influence on the HBE. However, this small shift is negligible compared with the pH effect that can cause as large as 0.15 eV shift when the pH changes from 0 to 13. It appears that the solution pH predominantly determines the HBE while other anions play a minor role. Figure 3: CVs and HBEs of Pt in a full range of solution pH. ( a ) Steady state CVs of Pt collected in selected Ar-saturated electrolytes at a sweep rate of 50 mV s −1 . The CV curves have been corrected for solution resistance. ( b ) HBEs on Pt(110) (solid symbols) and (100) (empty symbols) surfaces obtained from CVs as a function of solution pH. Error bars are s.d. of at least two sets of experimental repeats. Full size image The HOR/HER in acid is believed to go through either the Tafel–Volmer or Heyrovsky–Volmer sequence: In strong base, Durst et al . [22] suggest that the sequence does not change except that the Heyrovsky or Volmer step is followed by quick recombination between H + cations and abundant OH − anions in the alkaline electrolytes, and thus HBE is the dominating factor for the HOR/HER in both strong acid and strong base. The monotonic correlations between HBE and solution pH, as well as that between the HOR/HER rate and solution pH in multiple buffers and a much wider pH range shown in our study suggest that the HBE governs the HOR/HER activities in a full range of solution pHs. We plot the half-wave potential of the HOR and the overpotential of the HER at −1 mA cm −2 disk as a function of HBE in Fig. 4 , and exchange current density estimated using relation ( Supplementary Fig. 2 ) as a function of HBE in Supplementary Fig. 4 . As the HBE becomes stronger, the HOR half-wave potential and HER overpotential monotonically increase. Previous study and our data strongly support the hypothesis that the HBE is the sole factor governing the HOR/HER. A recent study of the HOR in alkaline environment shows that PtRu NPs exhibit a factor of 2 enhancement of HOR activity compared with Pt NPs [33] . The improvement of the HOR activity has been ascribed to the weakened HBE of PtRu relative to Pt, suggesting that tuning the HBE through alloying Pt with a second metal can be an effective approach for more efficient HOR electrocatalysis. So far, there is no direct evidence as to OH adsorption at potential as low as near the HOR/HER reversible potential, which is critical in the bifunctional mechanism proposed recently, stating that the co-existence of adsorbed H and OH would promote the reaction rate [20] , [23] . Here we propose that, instead of adsorbing to the Pt surface to promote the reaction, OH − in the solution phase more likely affects the HOR/HER activities through tuning the HBE. Although various anions have been used in the current study, the effect of which remains inconclusive, the alkalinity ( ) seems to be the major descriptor for the HBE as shown in Fig. 3 . Previous studies on the correlation between the HER and HBE have been established on DFT-calculated HBE values, which do not consider the effect from water or anions [2] , [11] . However, this solution effect may be very critical. A change of 13 units in pH could change the HBE by 0.15 eV, which in turn changes the HOR/HER activity by two orders of magnitude. 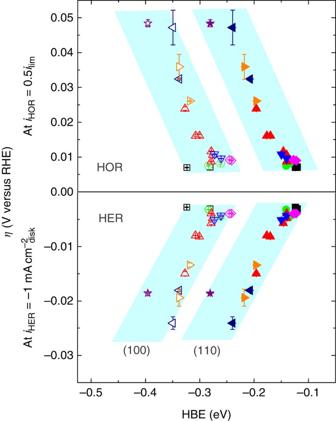Figure 4: Overpotential of the HOR/HER on Pt as a function of the HBE. The overpotential for the HOR is ati=0.5ilimand the overpotential for the HER is ati=−1 mA cm−2diskin all pH-buffered electrolytes on Pt(110) (solid symbols) and (100) (open symbols) surfaces. Error bars are s.d. of at least two sets of experimental repeats. Figure 4: Overpotential of the HOR/HER on Pt as a function of the HBE. The overpotential for the HOR is at i =0.5 i lim and the overpotential for the HER is at i =−1 mA cm −2 disk in all pH-buffered electrolytes on Pt(110) (solid symbols) and (100) (open symbols) surfaces. Error bars are s.d. of at least two sets of experimental repeats. Full size image In summary, our study of HOR/HER in pH-buffered electrolytes reveals that HBE is likely the sole descriptor for the HOR/HER activities on single metallic Pt. The experimentally measured HBE of Pt is determined from CVs and found to increase with pH, while the HOR/HER activity decreases with pH. We propose that the OH species do not directly participate in the reactions through adsorption, while the alkalinity (OH − in the solution phase) changes the HBE and in turn influences the HOR/HER activity. It is of great interest and importance to unravel the fundamentals behind the correlation between the HBE and the solution alkalinity. Furthermore, this finding highlights the significance of solution pH for designing HOR/HER electrocatalysts under different application environments. Preparation of electrolytes 0.1 and 1 M perchloric acid (HClO 4 ), 0.1 M and 1 M sulfuric acid (H 2 SO 4 ), 0.1 M and 0.2 M phosphoric acid (H 3 PO 4 ), 0.1 M potassium hydroxide (KOH), 0.2 M acetic acid (CH 3 COOH), 0.2 M citric acid (C 6 H 8 O 7 ), 0.2 M boric acid (H 3 BO 3 ) and 0.2 M potassium bicarbonate (KHCO 3 ) were prepared by dissolving HClO 4 (concentration of 70%, EMD), H 2 SO 4 (95%, EMD), H 3 PO 4 (99.99% Sigma Aldrich), KOH pellets (99.99% metal trace, Sigma Aldrich), CH 3 COOH (99.9% Fisher Scientific), C 6 H 8 O 7 (99% Sigma Aldrich), H 3 BO 3 (99% Alfa Aesar) and KHCO 3 (99.7% Sigma Aldrich) in deionized water (18.2 MΩ cm). Buffer solution electrolytes were made by adding 2, 4, 6, 8 and 10 ml of ~3.7 M KOH to each 100 ml of 0.2 M H 3 PO 4 solution, 2 ml and 4 ml of ~3.7 M KOH to each 100 ml of 0.2 M CH 3 COOH, 100 ml of 0.2 M C 6 H 8 O 7 , 100 ml of 0.2 M H 3 BO 3 and 100 ml of 0.2 M KHCO 3 solutions, respectively. All chemicals were used as received without further purification. Electrochemical measurements Electrochemical measurements were performed in a one-compartment glass cell (Pine Ins. ), with polycrystalline Pt disk (5 mm in diameter, Pine Ins.) mounted on a rotator (Pine Ins.) as the working electrode and a spiral Pt wire (Pine Ins.) as the counter electrode. Before use, the Pt disk was polished with 1 and 0.05 μm alumina polishing slurries and cleaned with deionized water. A saturated calomel electrode (SCE, Princeton Applied Research), as the reference electrode, was immersed in a Luggin capillary (Princeton Applied Research) filled with 2 M potassium nitrate (KNO 3 , Sigma Aldrich) solution, which serves as the salt bridge to (1) minimize the junction potentials at the interfaces, (2) prevent Cl − in the SCE from contaminating the investigated electrolytes and (3) maintain a stable SCE potential in an alkaline environment. The detail of the SCE stability was described in Supplementary Note 3 and Supplementary Fig. 5 . All potentials were reported on a reversible hydrogen electrode scale. CVs of Pt were collected after the electrolytes were saturated with Argon (Ar). A few fast scans (200 mV s −1 ) were applied to remove the surface contaminants if needed. Steady state CVs at a scanning rate of 50 mV s −1 were recorded. Hydrogen adsorption/desorption region in CV collected in 0.1 M HClO 4 electrolyte was used to determine the electrochemical surface area of the Pt disk. The electrochemical surface area of Pt was calculated to be 0.42 cm 2 Pt , assuming a charge density of 210 μC cm −2 Pt for one monolayer of H adsorption [34] . The roughness factor A rf was calculated to be 2.1. HOR/HER were performed in H 2 -saturated electrolytes at a rotating speed of 1,600 r.p.m. The HER current densities were controlled not to exceed −2 mA cm −2 disk to minimize H 2 bubble accumulation. Steady state polarization curves at 10 mV s −1 were recorded for comparison. Solution resistances ( R ) were measured using the a.c.-impedance spectroscopy method. The a.c.-impedance spectra were collected from 200 kHz to 100 mHz at a constant potential with a 10 mV potential perturbation. All of the i–E curves reported in this paper were corrected for solution resistance using E=E measured −iR . Determination of solution pH Solution pH values were calculated from the HOR/HER reversible potential (versus SCE), which follows the Nernst equation. At 0 A HOR/HER current, the surface pH is essentially the pH of the bulk solution. The potential where the current is 0 A, and the pH satisfy the following equation: where is the HOR/HER reversible potential (equivalent to open circuit voltage, OCV) versus SCE, and E SCE is the standard SCE potential. How to cite this article : Sheng, W. et al . Correlating hydrogen oxidation and evolution activity on platinum at different pH with measured hydrogen binding energy. Nat. Commun. 6:5848 doi: 10.1038/ncomms6848 (2015).